Covalency does not suppress O2formation in 4d and 5d Li-rich O-redox cathodes 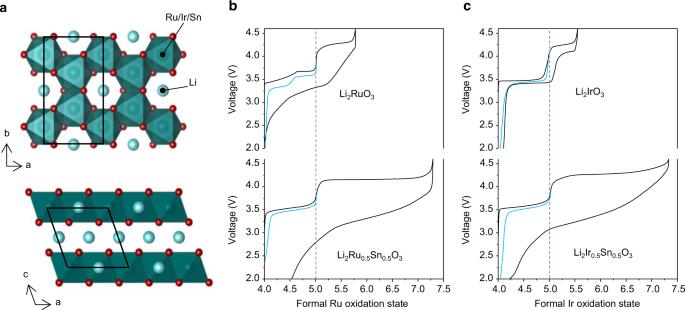Fig. 1: Structure and electrochemistry of Li-rich 4d- and 5d-based cathodes. aO3-type layered structure with honeycomb ordering of Li and TM ions within the TM layers. First cycle load curves forbLi2RuO3and Li2Ru0.5Sn0.5O3and (c) Li2IrO3and Li2Ir0.5Sn0.5O3from 2.0 V to 4.6 V at a current rate of 20 mA g−1plotted against formal oxidation state of Ru or Ir (in black). Electrochemical cycling is reversible with little voltage hysteresis below +5 (in blue). High voltage charging plateaus are observed in all materials beyond the +5 TM oxidation state. The plateaus are accompanied by significant voltage loss on subsequent discharge in all cases except for Li2IrO3. Layered Li-rich transition metal oxides undergo O-redox, involving the oxidation of the O 2− ions charge compensated by extraction of Li + ions. Recent results have shown that for 3d transition metal oxides the oxidized O 2− forms molecular O 2 trapped in the bulk particles. Other forms of oxidised O 2− such as O 2 2− or (O–O) n− with long bonds have been proposed, based especially on work on 4 and 5d transition metal oxides, where TM–O bonding is more covalent. Here, we show, using high resolution RIXS that molecular O 2 is formed in the bulk particles on O 2‒ oxidation in the archetypal Li-rich ruthenates and iridate compounds, Li 2 RuO 3 , Li 2 Ru 0.5 Sn 0.5 O 3 and Li 2 Ir 0.5 Sn 0.5 O 3 . The results indicate that O-redox occurs across 3, 4, and 5d transition metal oxides, forming O 2 , i.e. the greater covalency of the 4d and 5d compounds still favours O 2 . RIXS and XAS data for Li 2 IrO 3 are consistent with a charge compensation mechanism associated primarily with Ir redox up to and beyond the 5+ oxidation state, with no evidence of O–O dimerization. Layered Li-rich 3d transition metal oxide intercalation compounds, such as Li[Li 0.2 Ni 0.13 Co 0.13 Mn 0.54 ]O 2 , have received a great deal of attention because Li + can be extracted beyond the limit of transition metal (TM) oxidation, with the charge being compensated by oxidation of the O 2‒ ions (O-redox) [1] , [2] , [3] , [4] , [5] , [6] , [7] , [8] , [9] . These compounds typically possess honeycomb ordered Li and TM within the TM layer. However, Mn-based honeycomb ordered structures do not provide a stable framework for oxidised O 2− and have been shown to undergo extensive TM migration, and bulk O–O dimerization leading to voltage hysteresis and loss of energy density, in addition to surface O 2 evolution [10] , [11] , [12] , [13] , [14] . It has been shown recently that the dimerised O–O is molecular O 2 , which is trapped in voids within the bulk of the charged particles [15] , [16] . Molecular O 2 formation is responsible for both surface O-loss and bulk O-redox. Pioneering work by Tarascon, Doublet and co-workers [17] , [18] , [19] , [20] , [21] , [22] , [23] , [24] , [25] and by others [26] , [27] , [28] , [29] , [30] , [31] , on the 4d- and 5d-based analogues of the 3d compounds, such as Li 2 RuO 3 , Na 2 RuO 3 , Li 2 Ru 0.5 Mn 0.5 O 3 , Li 2 IrO 3 and Li 2 Ir 0.75 Sn 0.25 O 3 , has led to important advances in the understanding of O-redox. These systems possess the same honeycomb ordered Li and TM ions within the TM layer. With the exception of Li 2 IrO 3 , they exhibit voltage hysteresis, with a plateau on charge and a low voltage S-shaped profile on subsequent discharge. Loss of honeycomb ordering due to Li/TM disordering accompanies the voltage hysteresis along with O 2 loss from the surface of the particles [17] , [19] , [21] , [26] , [29] . It has been reported that peroxides O 2 2− and longer O–O dimers form beyond the limits of transition metal oxidation in the 4 and 5d transition metal oxides [17] , [19] . The more strongly hybridised TM–O bonding of the 4 and 5d transition metals compared with the 3d counterparts has been cited as a reason for stabilising such O–O species with longer O–O bonds [18] , [19] , [20] , [32] . In highly covalent transition metal sulphides, selenides and tellurides, electron holes can be stabilised through dimerization of the chalcogen (S 2 ) 2− which remains coordinated to the transition metal due to the strong orbital overlap [33] . It has proved very challenging to identify experimentally the form of oxidised O 2− in charged materials. The recent application of high resolution RIXS spectroscopy has proved useful in probing the nature of oxidised O 2− [15] , [16] . Here we apply this technique to the 4 and 5d materials, providing direct evidence for the presence of molecular O 2 , trapped in the bulk of the archetypal 4d and 5d systems Li 2 RuO 3 , Li 2 Ru 0.5 Sn 0.5 O 3 and Li 2 Ir 0.5 Sn 0.5 O 3 . The O 2 is formed only through charging across the high voltage plateau and is reduced on subsequent discharge, in line with our findings for Li 1.2 Ni 0.13 Co 0.13 Mn 0.54 O 2 , disordered rocksalt Li 2 MnO 2 F and the P2-type Na-ion cathodes [15] , [16] , [34] . We find no evidence of molecular O 2 formation or other O–O dimers in Li 2 IrO 3 up to the limits of oxidation and instead identify stable electron holes formed in bonding TM–O orbitals, consistent with previous reports indicating reversible Ir 5+ to Ir 5.5+ oxidation instead of O oxidation and reinforcing the link between bulk O 2 formation and the loss of high voltage plateau [26] . These data indicate that the more covalent TM–O bonding in 4 and 5d compared with 3d TM oxides still favours the formation of molecular O 2 , helping to explain why O-loss is also observed from the surface of these compounds. 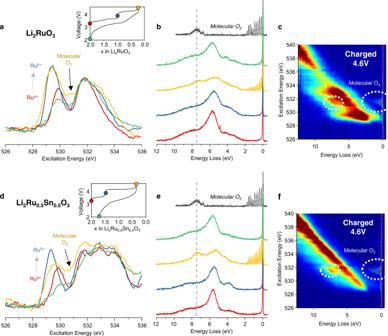Fig. 2: O XAS and RIXS spectroscopy for Li-rich ruthenates. a,dO K-edge XAS spectra collected in bulk sensitive partial fluorescence yield (PFY) mode. Inset figure—load curve showing with coloured dots where on the load curve the spectra were collected.b,ehigh resolution RIXS line scans at an excitation energy of 531 eV. Spectrum of molecular O2gas shown for reference in black (reproduced from ref.35). The RIXS line scans reveal the formation of molecular O2which is reduced to O2−on discharge.c,fHigh resolution RIXS maps of the O K-edge pre-edge for cathodes charged to the end of the high voltage plateau. Across the plateau there is an increase in area at 531 eV for both Li2RuO3and Li2Ru0.5Sn0.5O3. The RIXS maps show that there are no other O–O vibrations. The implication is that the O-redox process, involving molecular O 2 formation at the surface and in the bulk, is the same for Li-rich systems with the honeycomb superstructure moving down the Periodic Table. The Li-rich ruthenates and iridates Li 2 RuO 3 , Li 2 IrO 3 and Sn-substituted Li 2 Ru 0.5 Sn 0.5 O 3 and Li 2 Ir 0.5 Sn 0.5 O 3 were prepared following the methods of previous reports [17] , [19] . Powder X-ray Diffraction data, Supplementary Figs. 1 – 3 , confirm the formation of the compounds. Each of the materials possess O3-type layered structures with honeycomb ordering in the TM plane, Fig. 1a manifesting as the familiar superlattice peaks between 2θ = 18° and 34°. As seen before, there is evidence of some stacking faults between the ordered layers, which result in asymmetric peak broadening of these superlattice peaks, especially for the Sn-substituted samples. Fig. 1: Structure and electrochemistry of Li-rich 4d- and 5d-based cathodes. a O3-type layered structure with honeycomb ordering of Li and TM ions within the TM layers. First cycle load curves for b Li 2 RuO 3 and Li 2 Ru 0.5 Sn 0.5 O 3 and ( c ) Li 2 IrO 3 and Li 2 Ir 0.5 Sn 0.5 O 3 from 2.0 V to 4.6 V at a current rate of 20 mA g −1 plotted against formal oxidation state of Ru or Ir (in black). Electrochemical cycling is reversible with little voltage hysteresis below +5 (in blue). High voltage charging plateaus are observed in all materials beyond the +5 TM oxidation state. The plateaus are accompanied by significant voltage loss on subsequent discharge in all cases except for Li 2 IrO 3 . Full size image The first cycle load curves are shown in Fig. 1b, c and are plotted against the nominal oxidation state of Ru and Ir in each case, since Sn 4+ is known to be redox inactive. The electrochemical behaviour is reversible with very little hysteresis when cycling below Ru 5+ and Ir 5+ . When sufficient Li is extracted to exceed the +5 oxidation state on Ru, an extended high voltage plateau is observed followed by an S-shaped discharge. For the iridates, reversibility can be maintained up to +5.5 supported by Ir redox as shown recently by Hong et al. [26] . Further Li can be extracted beyond this limit in Li 2 Ir 0.5 Sn 0.5 O 3 subsequently inducing voltage hysteresis. Li 2 IrO 3 is the only material where TM migration and loss of the honeycomb ordering is avoided upon charging to 4.6 V, in accord with its reversible electrochemical behaviour [26] , [30] . Spectroscopic characterisation of O Understanding O-redox has proven to be a challenge due in part to the need for techniques capable of determining the nature of O species formed in the bulk. In this study, we have employed X-ray absorption spectroscopy (XAS) in partial fluorescence yield (PFY) mode and high resolution resonant inelastic X-ray scattering (RIXS) at the O K-edge, as they offer a direct probe of the electronic states on O at depths of up to 50–100 nm into the sample. XAS probes the empty states above the Fermi level. In RIXS, excitation of core electrons to empty states above the Fermi level results in emission as electrons from filled valance states below the Fermi level relax to the core-hole states. 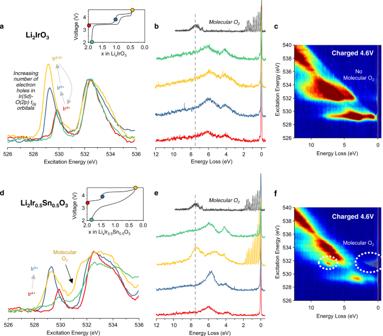Fig. 3: O XAS and RIXS spectroscopy of Li-rich iridates. a,dO K-edge XAS spectra collected in bulk sensitive partial fluorescence yield (PFY) mode. Inset figure—load curve showing with coloured dots where on the load curve the spectra were collected.b,eHigh resolution RIXS line scans at an excitation energy of 531 eV. Spectrum of molecular O2gas shown for reference in black (reproduced from ref.35). The RIXS line scans reveal the formation of molecular O2in Li2Ir0.5Sn0.5O3which is reduced to O2−on discharge but not in Li2IrO3.c,fHigh resolution RIXS maps of the O K-edge pre-edge for cathodes charged to the end of the high voltage plateau. The RIXS maps show that there are no other vibrations. RIXS complements XAS as it provides a direct probe of the valence states on O. In Fig. 2 , we present the O K-edge XAS and RIXS for Li 2 RuO 3 and Li 2 Ru 0.5 Sn 0.5 O 3 collected ex situ at different points along the load curve on charge and discharge. Considering first the XAS spectra. For Li 2 RuO 3 , on initial charge to the beginning of the plateau, there is a pronounced increase in intensity at the leading edge of the pre-edge (lowest energy peak between 529 and 530 eV) indicating the formation of electron hole states in hybridised Ru–O orbitals consistent with Ru oxidation from +4 to +5, as previously reported [17] , [25] . Across the plateau there is no further increase in this region but instead new states appear at 531 eV. After discharge, both of these changes are reversed, and the pre-edge reduces in intensity. The pre-edge for the discharged sample is comparatively broad when compared directly with that of the pristine indicating a rehybridization of the Ru–O bonding between the two samples. The structure has been shown to undergo TM migration during the first cycle and the XAS peak broadening we observe here is consistent with an increase in the local disorder around O. For Li 2 Ru 0.5 Sn 0.5 O 3 , the pre-edge broadening after the plateau on charge and in the discharged material is more pronounced than Li 2 RuO 3 in line with the greater degree of O-redox and more extensive TM migration for the Sn-substituted material [17] . Fig. 2: O XAS and RIXS spectroscopy for Li-rich ruthenates. a , d O K-edge XAS spectra collected in bulk sensitive partial fluorescence yield (PFY) mode. Inset figure—load curve showing with coloured dots where on the load curve the spectra were collected. b , e high resolution RIXS line scans at an excitation energy of 531 eV. Spectrum of molecular O 2 gas shown for reference in black (reproduced from ref. [35] ). The RIXS line scans reveal the formation of molecular O 2 which is reduced to O 2− on discharge. c , f High resolution RIXS maps of the O K-edge pre-edge for cathodes charged to the end of the high voltage plateau. Across the plateau there is an increase in area at 531 eV for both Li 2 RuO 3 and Li 2 Ru 0.5 Sn 0.5 O 3 . The RIXS maps show that there are no other O–O vibrations. Full size image To interrogate the electronic states formed at 531 eV further, RIXS measurements were performed for each sample at this excitation energy. The emission spectra are plotted as is convention, as energy loss (difference between excitation and emission energy). At the top of charge two new energy loss features become evident, a broad peak at 8 eV and a progression of sharp peaks between 0 and 2 eV, as we observed previously for Li 1.2 Ni 0.13 Co 0.13 Mn 0.54 O 2 and Na 0.75 Li 0.25 Mn 0.75 O 2 [15] , [16] . The progression of peaks in the 0–2 eV region correspond to the vibrations of a molecular O 2 diatomic, also shown in Fig. 2 [35] . The emission spectra for a range of excitation energies across the O K-edge for the fully charged electrodes were also measured and are presented as RIXS maps. The data show no evidence of any other vibrational features at different excitation energies. After discharge, these new features are much diminished in intensity indicating reversible electrochemical reduction of molecular O 2 has occurred. The same measurements were also performed for the iridate samples and are presented in Fig. 3 . Li 2 Ir 0.5 Sn 0.5 O 3 exhibits very similar changes to those described for Li 2 RuO 3 and Li 2 Ru 0.5 Sn 0.5 O 3 consistent with the voltage profile observed. On the other hand, the RIXS spectra for Li 2 IrO 3 do not show any evidence for the presence of molecular O 2 in the fully charged electrodes. Instead, a strong increase in intensity at the leading edge of the pre-edge is seen when charging Ir beyond the +5 oxidation state. This observation supports the conclusion that the high voltage plateau in Li 2 IrO 3 is associated with Ir rather than O oxidation [26] . Notably, the XAS spectra for the pristine and discharged electrodes are almost fully superimposable indicating minimal irreversible change to the electronic structure and thus structural stability. Fig. 3: O XAS and RIXS spectroscopy of Li-rich iridates. a , d O K-edge XAS spectra collected in bulk sensitive partial fluorescence yield (PFY) mode. Inset figure—load curve showing with coloured dots where on the load curve the spectra were collected. b , e High resolution RIXS line scans at an excitation energy of 531 eV. Spectrum of molecular O 2 gas shown for reference in black (reproduced from ref. [35] ). The RIXS line scans reveal the formation of molecular O 2 in Li 2 Ir 0.5 Sn 0.5 O 3 which is reduced to O 2− on discharge but not in Li 2 IrO 3 . c , f High resolution RIXS maps of the O K-edge pre-edge for cathodes charged to the end of the high voltage plateau. The RIXS maps show that there are no other vibrations. Full size image Since the measurements are performed under ultra-high vacuum (UHV) conditions and the samples had been pumped down overnight under UHV, the electrodes will be fully out-gassed, so any molecular species that are detected are trapped within the bulk of the primary particles. To rule out the possible influence of beam damage inducing molecular O 2 , we performed all our measurements at low temperature, 20 K, and conducted measurements at the same sample location over a range of timescales. The data presented in Supplementary Fig. 4 show no change in the peak spacing between spectra acquired after 30 s and 1800 s exposure times and only a minor decrease in intensity, which is in line with our previous beam sensitivity studies for molecular O 2 in Li 1.2 Ni 0.13 Co 0.13 Mn 0.54 O 2 [15] . In that paper, we also extensively examined the effect of temperature and photon flux and showed that neither of these factors have a detectable influence on the vibrational peak spacing, reinforcing that the O 2 observed by RIXS is intrinsic to the cathode. Although the spectroscopic data show no evidence of O species other than O 2 , RIXS data were also collected for KO 2 and Li 2 O 2 to rule out the possibility of O 2− and O 2 2− . The results are presented in Fig. 4 where they are compared directly with the spectra for the Ru and Ir compounds. The peak spacing for Li 2 O 2 around the elastic peak corresponding to the vibrational spectrum is almost exactly half of the peak spacing observed for molecular O 2 in the cathodes as clearly seen in the Birge-Sponer plot, Fig. 4b . This is closely in line with the vibrational frequency for O 2 2− which is well known to be half that of molecular O 2 . For KO 2 , containing the superoxide moiety O 2 − of intermediate bond order to O 2 and O 2 2− , the peak spacing lies halfway between the two. While some differences in the RIXS spectra for different peroxide and superoxide compounds is possible, the vibrational spectra associated with the elastic peak is determined primarily by the O–O bond length/strength and therefore is characteristic of these species in general. The clear distinction that can be made between O 2 , O 2 − and O 2 2− dimers demonstrates the power of high resolution RIXS and provides evidence for the formation of molecular O 2 in the Li-rich cathodes. Fig. 4: Direct spectroscopic evidence against peroxides in charged 4d and 5d cathodes. a High resolution RIXS scans at 531 eV excitation energy for charged cathode samples and a Li 2 O 2 reference collected under identical measurement conditions. KO 2 RIXS was collected at 529.6 eV, where O 2 − vibrations are strongest. Peak spacing consistent with molecular O 2 is seen in the case of all cathodes except Li 2 IrO 3 which is not O-redox active. There is no evidence of O 2 2− or O 2 − vibrations in any of the cathode samples ruling out the presence of peroxides and superoxides. b Birge-sponer plot showing linearly decreasing dependence of peak spacing with vibrational quantum number, n , consistent with the anharmonic oscillations of diatomic molecules. Full size image Studies using X-ray photoelectron spectroscopy (XPS), electron paramagnetic resonance (EPR) and density functional theory (DFT) pointed to the possibility of peroxo-like O 2 n− species, where n = 1, 2 or 3 [17] , [20] , [25] , [36] . Scanning transmission spectroscopy (STEM) and neutron powder diffraction studies of Li 2 IrO 3 , suggested longer peroxo-like dimers (3 < n < 3.3) [19] . However, excellent though these studies are, it is a challenge for these techniques to identify unambiguously the nature of the oxidised oxygen species. XPS, being an electron emission technique, is, in general, more limited in its ability to measure bulk species than RIXS, which utilises photon emissions, and XPS can often be strongly influenced by surface contributions. Turning to local structural probes, imaging individual O–O defects in the bulk is beyond the capabilities of current STEM techniques and resolving O–O species at such low interatomic separations and concentrations is very challenging for total scattering data. Since they are magnetically complex materials, the 4d and 5d systems defy clear characterisation of oxidised O by either 17 O NMR or SQUID. In contrast, the high resolution RIXS that we employ in this study is element specific, probes 50–100 nm deep into the particles, and has allowed us to clearly identify molecular O 2 in the bulk of solid materials. High resolution RIXS has already provided evidence that O 2− oxidation in 3d TM oxides forms molecular O 2 trapped in voids in the bulk particles. This observation is further supported by 17 O NMR which not only identifies trapped molecular O 2 as the O–O species formed on charge, but also shows that it is present in quantities commensurate with that expected from the charged passed in Li 1.2 Ni 0.13 Co 0.13 Mn 0.54 O 2 [15] . Our RIXS and XAS results indicate that the O-redox process can be described as molecular O 2 formation throughout the cathode, both as evolved O 2 at the surface, which has already been demonstrated with operando mass spec [19] , [29] , and trapped O 2 within the bulk. The 4 and 5d transition metal oxides generally exhibit greater covalency in the TM–O bond than those of their 3d counterparts; associated with the greater TMd-O2p overlap and lower electron repulsion of the larger 4 and 5d orbitals. The results presented here indicate that these more covalent systems bear closer resemblance to the 3d Li-rich materials than previously thought and that any greater covalency in the TM–O bond for 4 and 5d compounds does not suppress molecular O 2 formation in favour of other O–O species. In a recent study, Hong et al. presented Ir L 3 XANES data that showed Ir is able to oxidise beyond +5 to +5.5 in Li 2 IrO 3 and Li 2 Ir 0.5 Sn 0.5 O 3 before O-redox activity [26] . In this regime, both materials can cycle reversibly. For Li 2 Ir 0.5 Sn 0.5 O 3 , charging can be continued beyond +5.5 consequently incurring O oxidation, TM migration, peroxide (O 2 2− ) formation and voltage hysteresis. Our results show an absence of any oxidised oxygen species in Li 2 IrO 3 in accord with the Ir L 3 XANES data presented by Hong et al [26] . However, for Li 2 Ir 0.5 Sn 0.5 O 3 the high resolution RIXS shows the presence of molecular O 2 , rather than peroxide, as the only form of oxidised oxygen species. High resolution RIXS also reveals molecular O 2 is present in the ruthenates in contrast to previous reports of peroxides. The ability of RIXS to show an absence of signal for materials supported exclusively by TM-redox and identify oxidised O when it is present in O-redox materials demonstrates its utility for probing oxidised O species. Ir 5+ , low spin t 2g 4 , has 1 more electron than Ru 5+ , t 2g 3 , and it is spin-paired, Fig. 5a . Removal of this higher energy spin down electron occurs at a lower voltage than for an electron on Ru 5+ . The oxidation of O 2− sits between the energies for Ir 5+/6+ and Ru 5+/6+ such that Ir 5+ is oxidised before O 2− (i.e. at a lower voltage) whereas Ru 5+ is not. The voltages of the redox couples derived from dQ/dV analysis of the electrochemical load curves in Fig. 1 are shown in Fig. 5b . The substitution of Ir for Sn limits the Ir redox capacity increasing the amount of extractable Li available to be charge compensated by O-redox explaining why substantial O oxidation is observed for Li 2 Ir 0.5 Sn 0.5 O 3 . Fig. 5: Redox potentials. a d electron configurations for different oxidation states of Ru and Ir. The spin down electron on Ir 5+ is at a higher energy and hence oxidised at a lower voltage than removal of a spin up electron from the stable d 3 configuration of Ru 5+ . Since oxidation of Ir 5+ occurs before O 2− /O 2 and Ru 5+ does not, we place O 2− /O 2 between the two redox couples in the figure ( b ). The values of the redox couples shown in black in ( b ) were obtained from dQ/dV analysis extracted from the data in Fig. 1 . Full size image Much like the 3d TM Li-rich O-redox systems, those based on 4d and 5d TM elements exhibit TM migration, loss of honeycomb ordering, O-loss and voltage hysteresis. The vibrational spectra measured by RIXS now also show that molecular O 2 , rather than peroxides or peroxo-like species, are formed in all of these systems indicating TM–O covalency has limited effect on the bond order of the O–O dimer in the bulk of the cathodes. Future research efforts on Li-rich cathodes should focus on chemical and structural modifications other than covalency of the host network to improve their performance. Materials preparation Li 2 RuO 3 and Li 2 Ru 0.5 Sn 0.5 O 3 were synthesised from RuO 2 (99.9% Alfa Aesar), SnC 2 O 4 (98% Alfa Aesar) and Li 2 CO 3 (99+% Merck) mixed in the appropriate ratios with 10% excess Li 2 CO 3 . Calcination was performed in air at 800 °C for 6 h, 900 °C for 12 h and then 1100 °C for 12 h with intermediate grinding. Li 2 IrO 3 and Li 2 Ir 0.5 Sn 0.5 O 3 were synthesised from IrO 2 (99.9% Alfa Aesar), SnO 2 (99.9% Alfa Aesar) and Li 2 CO 3 (99+% Merck) mixed in the appropriate ratios with 10% excess Li 2 CO 3 . Calcination was performed in air at 1000 °C for 12 h and 900 °C for 36 h with intermediate grinding. The as-prepared materials were transferred to an Ar-filled glovebox and handled under inert atmosphere for all further manipulations. Li 2 O 2 (95%, ACROS Organics) and KO 2 (Sigma Aldrich) standards were used as supplied. Electrochemistry Self-supporting electrode films were prepared by grinding the as-synthesised materials with acetylene black and polytetrafluoroethylene in a 8:1:1 mass ratio in a pestle and mortar and subsequently calendared. Electrochemical cycling was performed in coin cells with LP30 electrolyte and a lithium metal foil counter electrode. Cells were disassembled at different states of charge and the electrodes rinsed with dry dimethylcarbonate for ex situ analysis. Powder X-ray diffraction Powder X-ray diffraction patterns were obtained for the as-prepared materials using a Cu source Rigaku SmartLab diffractometer equipped with a Ge(220) double bounce monochromator and without exposure to air. Reitveld profile refinements were performed using the GSAS suite of programs. X-ray absorption spectroscopy and resonant inelastic X-ray scattering X-ray absorption spectroscopy and resonant inelastic X-ray scattering data were obtained at the I21 beamline, Diamond Light Source. Samples were transferred to the spectrometer using a vacuum transfer suitcase to avoid air exposure and were pumped down to UHV and left to fully degas overnight. O K-edge spectra were obtained in partial fluorescence mode for bulk sensitivity. RIXS line scans were recorded at five different sample locations and averaged together. RIXS maps were collected at 0.2 eV intervals in excitation energy. 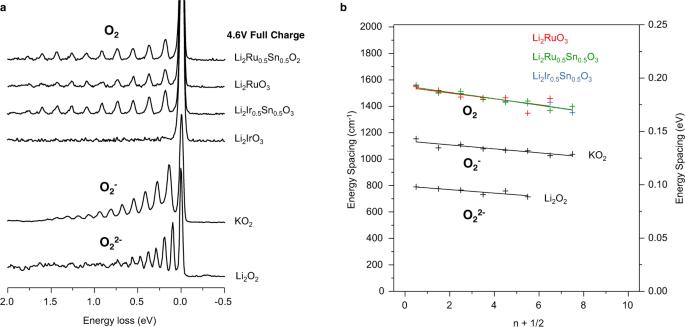Fig. 4: Direct spectroscopic evidence against peroxides in charged 4d and 5d cathodes. aHigh resolution RIXS scans at 531 eV excitation energy for charged cathode samples and a Li2O2reference collected under identical measurement conditions. KO2RIXS was collected at 529.6 eV, where O2−vibrations are strongest. Peak spacing consistent with molecular O2is seen in the case of all cathodes except Li2IrO3which is not O-redox active. There is no evidence of O22−or O2−vibrations in any of the cathode samples ruling out the presence of peroxides and superoxides.bBirge-sponer plot showing linearly decreasing dependence of peak spacing with vibrational quantum number,n, consistent with the anharmonic oscillations of diatomic molecules. 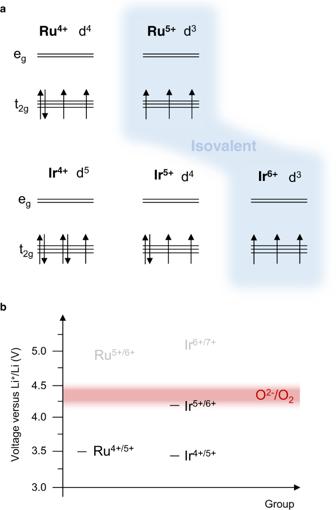Fig. 5: Redox potentials. ad electron configurations for different oxidation states of Ru and Ir. The spin down electron on Ir5+is at a higher energy and hence oxidised at a lower voltage than removal of a spin up electron from the stable d3configuration of Ru5+. Since oxidation of Ir5+occurs before O2−/O2and Ru5+does not, we place O2−/O2between the two redox couples in the figure (b). The values of the redox couples shown in black in (b) were obtained from dQ/dV analysis extracted from the data in Fig.1. All measurements were performed at 20 K to minimise any possible beam damage.